Southern Hemisphere control on Australian monsoon variability during the late deglaciation and Holocene The evolution of the Australian monsoon in relation to high-latitude temperature fluctuations over the last termination remains highly enigmatic. Here we integrate high-resolution riverine runoff and dust proxy data from X-ray fluorescence scanner measurements in four well-dated sediment cores, forming a NE–SW transect across the Timor Sea. Our records reveal that the development of the Australian monsoon closely followed the deglacial warming history of Antarctica. A minimum in riverine runoff documents dry conditions throughout the region during the Antarctic Cold Reversal (15–12.9 ka). Massive intensification of the monsoon coincided with Southern Hemisphere warming and intensified greenhouse forcing over Australia during the atmospheric CO 2 rise at 12.9–10 ka. We relate the earlier onset of the monsoon in the Timor Strait (13.4 ka) to regional changes in landmass exposure during deglacial sea-level rise. A return to dryer conditions occurred between 8.1 and 7.3 ka following the early Holocene runoff maximum. The response of the Australian monsoon to high-latitude temperature fluctuations on centennial to millennial timescales is still poorly understood due to the scarcity of continuous high-resolution precipitation records from Australia and Indonesia. Climate models predict drier subtropics in the Southern Hemisphere during interstadials [1] due to northward shift of the Intertropical Convergence Zone (ITCZ) during Northern Hemisphere warming (Bølling–Allerød (B–A), 15–12.9 ka) and intensification of the austral summer monsoon during Northern Hemisphere cooling (Heinrich Stadial 1 (HS1), 18–15 ka and the Younger Dryas (YD), 12.9–11.7 ka). However, model predictions of a hemispherical seesaw during the last glacial termination are not fully supported by climate proxy data, which are especially scarce for the Southern Hemisphere [2] , [3] , [4] . The evolution of the Australian monsoon during the B–A Northern Hemisphere warming and subsequent YD cooling events provides a test case to evaluate the impact of variations in the inter-hemispherical temperature gradient on tropical convective precipitation distribution. The B-A Northern Hemisphere warming occurred during a major cooling interval in Antarctica (Antarctic cold reversal, ACR), and the subsequent rapid austral warming at the end of the ACR resulted in the sharpest inter-hemispherical thermal gradient over the entire last glacial cycle [3] . This massive switch towards a warmer Southern Hemisphere was accompanied by a rapid rise in atmospheric CO 2 (ref. 5 ) that accentuated greenhouse forcing over the Australian continent, in a manner that matches scenarios of future climate change [6] . Here we combine X-ray fluorescence (XRF)-scanner-derived terrigenous river runoff and dust flux data in four well-dated sediment cores from the Timor Sea, which form a NE–SW transect across the southern front of the Indonesian–Australian monsoonal rain belt today ( Fig. 1 ; Supplementary Note 1 ; Supplementary Figs 1–3 ). This transect extends from an area dominated by river runoff from NW Australia (Fitzroy and Ord Rivers) to an area within the Timor Strait, with sedimentation dominated by runoff from monsoonal precipitation over Timor Leste and the southern Maluku islands. Terrigenous flux reconstructions are based on potassium (K) and aluminium (Al), which predominantly represent clay mineral-bound proxies for fine-grained riverine runoff [7] . We normalized K and Al against calcium (Ca), derived from biogenic carbonate, and against barium (Ba), related to the particulate organic matter flux and/or precipitation of barite by marine bacteria, inferring relatively small and independent variability in the flux rates of these two elements in relation to terrigenous flux ( Supplementary Figs 4–6 ). We quantified change points in the data series and provided uncertainty estimates using the software RAMPFIT, which was adapted to perform block bootstrap resampling [8] . We additionally used iron (Fe), titanium (Ti) and zirconium (Zr), which are elements enriched in aeolian dust from the NW Australian deserts in the southwestern Core SO185-18506, to track the northern limit of the NW Australian dust belt [9] . Our integrated data sets allow monitoring of secular variations in austral summer monsoonal runoff and austral winter aeolian dust fluxes originating from NW Australia over the last glacial termination and Holocene. Our records additionally provide a long-term perspective to evaluate the sensitivity of tropical rain belts to differential high-latitude warming in the Northern and Southern Hemispheres. In particular, our data show a major intensification of the Australian monsoon at 12.9–10 ka, which we relate to intensified greenhouse forcing over Australia during the deglacial atmospheric CO 2 rise, following rapid Southern Hemisphere warming. We attribute the earlier onset of the monsoon in the Timor Strait (13.4 ka) to regional changes in landmass exposure and cross-equatorial moisture transfer. Substantially dryer conditions returned throughout the region between 8.1 and 7.3 ka. 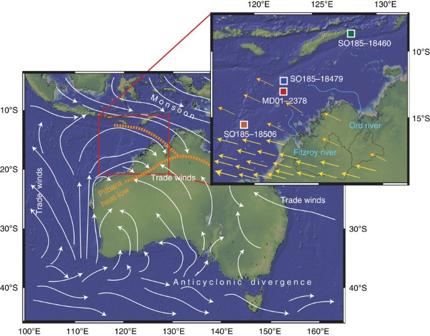Figure 1: Australian climate during the austral summer season. Heat low over the NW Australian Pilbara region and its eastward extension to the Kimberleys are indicated in orange. The basemap was generated with GeoMapApp (http://www.geomapapp.org) using the Global Multi-Resolution Topography synthesis database48. Yellow arrows on inset map indicate main aeolian dust paths8in September. Drainage Basins of Fitzroy and Ord Rivers49are marked with a black line. Approximate extension of the Fitzroy and Ord Rivers on the northwestern Australian shelf are indicated by blue dashed lines. Generalized wind patterns from ref.50. Position of cores investigated are shown in the inset map. Figure 1: Australian climate during the austral summer season. Heat low over the NW Australian Pilbara region and its eastward extension to the Kimberleys are indicated in orange. The basemap was generated with GeoMapApp ( http://www.geomapapp.org ) using the Global Multi-Resolution Topography synthesis database [48] . Yellow arrows on inset map indicate main aeolian dust paths [8] in September. Drainage Basins of Fitzroy and Ord Rivers [49] are marked with a black line. Approximate extension of the Fitzroy and Ord Rivers on the northwestern Australian shelf are indicated by blue dashed lines. Generalized wind patterns from ref. 50 . Position of cores investigated are shown in the inset map. Full size image Droughts in NW Australia during the ACR A salient feature of our fine-grained terrigenous records (ln(K/Ca)) is the spatial and temporal variability through the termination, except during the ACR and between 6 and 3 ka, when dry conditions generally prevailed throughout the region ( Fig. 2 ). The ACR is characterized by the lowest values in XRF-scanner-derived geochemical proxies for riverine input (ln(K/Ca) and ln((Al+K)/Ca) in Cores SO185-18506, MD01-2378 and SO185-18479, which are dominated by river runoff from NW Australia ( Fig. 2 ; Supplementary Note 1 ; Supplementary Fig. 1 ). The contribution of aeolian dust (ln(Zr+Ti+Fe)/(Al+K)) in Core SO185-18506 at the northern margin of the NW Australian ‘dust belt’ ( Figs 1 and 3 ) remains highly variable during the ACR, as during the Last Glacial Maximum (LGM) and HS1, in contrast to the early Holocene wet period. The lack of co-variance between the riverine and dust records prior to the YD probably relates to complex sediment-transport mechanisms due to lower sea-level and differential wind patterns. A regime of intense droughts during the ACR in NW Australia is also supported by recently published speleothem δ 18 O records from the Ball Gown Cave in NW Australia [10] ( Fig. 3 ). The remarkably dry conditions over NW Australia and the Timor Strait during the ACR bear strong similarity to the deglacial warming history of the Southern Hemisphere and Antarctica ( Fig. 2 ), which singles out the ACR as a distinct event, punctuating the otherwise continuous warming. 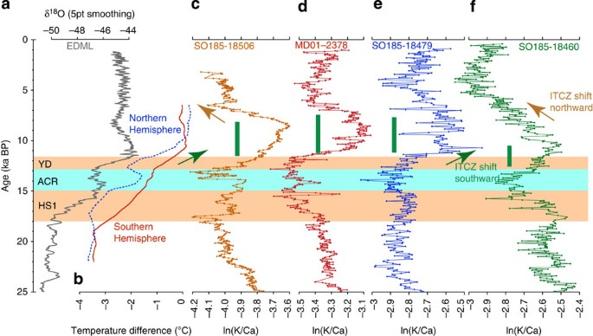Figure 2: XRF-scanner riverine runoff records from the Timor Sea. (a) EDML Antarctic ice core δ18Oicerecord51. (b) Northern and Southern Hemisphere temperature stacks3. (c) SO185-18506 (ln(K/Ca)). (d) MD01-2378 (ln(K/Ca)). (e) SO185-18479 (ln(K/Ca)). (f) SO185-18460 (ln(K/Ca)). HS1: Heinrich Stadial 1; ACR: Antarctic Cold Reversal; YD: Younger Dryas. Brown horizontal bands correspond to periods of Southern Hemisphere warming; light-blue horizontal band corresponds to a major cooling episode in Antarctica. ITCZ: Intertropical Convergence Zone. Green arrows indicate monsoon intensification associated with southward shift of ITCZ, brown arrows mark weakening of monsoon associated with northward shift of ITCZ. Green bars indicate monsoon maxima defined by change-points estimated using ramp-regression. Figure 2: XRF-scanner riverine runoff records from the Timor Sea. ( a ) EDML Antarctic ice core δ 18 O ice record [51] . ( b ) Northern and Southern Hemisphere temperature stacks [3] . ( c ) SO185-18506 (ln(K/Ca)). ( d ) MD01-2378 (ln(K/Ca)). ( e ) SO185-18479 (ln(K/Ca)). ( f ) SO185-18460 (ln(K/Ca)). HS1: Heinrich Stadial 1; ACR: Antarctic Cold Reversal; YD: Younger Dryas. Brown horizontal bands correspond to periods of Southern Hemisphere warming; light-blue horizontal band corresponds to a major cooling episode in Antarctica. ITCZ: Intertropical Convergence Zone. Green arrows indicate monsoon intensification associated with southward shift of ITCZ, brown arrows mark weakening of monsoon associated with northward shift of ITCZ. Green bars indicate monsoon maxima defined by change-points estimated using ramp-regression. 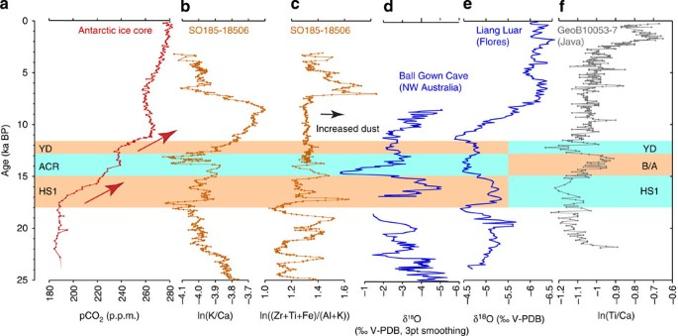Figure 3: Comparison of NW Australian and Indonesian precipitation and dust data. (a) Antarctic Ice Core (Dome Concordia) pCO2record5, red arrows indicate main phases of atmospheric pCO2increase. (b) XRF-scanner-derived riverine runoff from NW Australia (Core SO185-18506 ln(K/Ca)). (c) XRF-scanner-derived NW Australian aeolian dust proxy record (Core SO185-18506 ln((Zr+Ti+Fe)/(Al+K)). (d) NW Australian (Ball Gown Cave) speleothem δ18O precipitation record10. (e) Flores (Liang Luar) speleothem δ18O precipitation record17. (f) GeoB10053-7 ln(Ti/Ca) riverine runoff record off South Java14. ACR: Antarctic cold reversal; YD: Younger Dryas. Brown horizontal bands correspond to periods of Southern Hemisphere warming; light-blue horizontal band corresponds to a major cooling episode in Antarctica. Full size image Figure 3: Comparison of NW Australian and Indonesian precipitation and dust data. ( a ) Antarctic Ice Core (Dome Concordia) pCO 2 record [5] , red arrows indicate main phases of atmospheric pCO 2 increase. ( b ) XRF-scanner-derived riverine runoff from NW Australia (Core SO185-18506 ln(K/Ca)). ( c ) XRF-scanner-derived NW Australian aeolian dust proxy record (Core SO185-18506 ln((Zr+Ti+Fe)/(Al+K)). ( d ) NW Australian (Ball Gown Cave) speleothem δ 18 O precipitation record [10] . ( e ) Flores (Liang Luar) speleothem δ 18 O precipitation record [17] . ( f ) GeoB10053-7 ln(Ti/Ca) riverine runoff record off South Java [14] . ACR: Antarctic cold reversal; YD: Younger Dryas. Brown horizontal bands correspond to periods of Southern Hemisphere warming; light-blue horizontal band corresponds to a major cooling episode in Antarctica. Full size image Onset and early Holocene maximum of the Australian monsoon The onset of substantially wetter conditions after the ACR dry period occurred between 13.0 and 11.6 ka in the three cores off NW Australia ( Fig. 2 ). RAMPFIT-derived turning points for the ln(K/Ca) data sets are at 13.0 ±0.5 ka for Core SO185-18506, 11.6±0.2 ka for Core MD01-2378 and 12.5±0.4 ka for Core SO185-18479 ( Supplementary Figs 7–9 ). In the northeastern Core SO185-18460 within the Timor Strait, which is influenced by runoff from Timor and the southern Maluku islands, terrigenous flux started to increase earlier at 13.4±0.3 ka and continued to rise through the YD to a maximum between 12.5±0.3 and 10.5±0.4 ka ( Supplementary Figs 7–9 ; Supplementary Table 1 ). In contrast, the three cores receiving terrigenous supply from NW Australia show increases ~0.5–2 kyr later and exhibit a steep stepwise increase with consistent onset of the runoff maximum at 11.6±0.4 (SO185-18506), 11.2±0.2 (MD01-2378) and 11.1±0.4 ka (SO185-18479) ( Supplementary Figs 7–9 ). The structure of the runoff maximum also exhibits differences in the NW Australian margin cores and the Timor Strait core. Whereas Cores MD01-2378, SO185-18479 and SO185-18506 are characterized by relatively broad ln(K/Ca) plateaus between ~11.5 and ~8.0 ka, the precipitation maximum in the Timor Strait Core SO185-18460 is confined to a relatively short duration of ~2 kyr (RAMPFIT-derived turning points at 12.5±0.3 and 10.5±0.4 ka) at the base of the Holocene. An early Holocene precipitation maximum is also documented in pollen records [11] from a core located ~700 km south of Core SO185-18506, supporting the suggestion that the Australian summer monsoon extended as far as 22°S at that time. End of the early Holocene wet period The return to substantially dryer conditions, expressed by a decrease in ln(K/Ca), following the extended early Holocene runoff maximum was almost synchronous, occurring between 8.1 and 7.3 ka in the three cores off NW Australia ( Fig. 2 ; Supplementary Figs 7–9 ). However, the decrease in ln(K/Ca) starts earlier (10.5±0.4 ka) in the Timor Strait Core SO185-18460, which records runoff from Timor and the southern Maluku islands. The onset of a second runoff minimum occurs at 6.7±0.1 and 6.6±0.2 ka in the two most southwesterly cores off NW Australia (SO185-18506 and MD01-2378, respectively) and slightly later at 4.6±0.9 and 4.5±0.3 ka in the northern cores (SO185-18479 and SO185-18460, respectively). An abrupt, massive increase in ln((Zr+Ti+Fe)/(Al+K)) at 7.0 ka in Core SO185-18506 ( Fig. 3 ) marks a substantial increase in aeolian dust, concomitant with the decrease in riverine input, indicating a northward shift of the West-Australian dust belt. The major intensification of the Australian monsoon over the Timor Sea and NW Australia, following the end of the ACR dry period, coincided with intense cooling of the Northern Hemisphere and rapid warming of the Southern Hemisphere [3] . Today, cold surges over the South China Sea during boreal winter act as a trigger of Australian summer monsoon by ‘pushing’ the ITCZ southwards, thus initiating and intensifying monsoonal rainfall over northern Australia [12] . To which degree Australian monsoon variability was controlled by rapid large-amplitude climate events in the Northern Hemisphere during the last glacial period is still debated, but there is growing evidence that massive high-latitude cooling during Heinrich Stadials and warming during subsequent warm events resulted in substantial southward (cooling) and northward (warming) displacement of the ITCZ [1] , [2] , [13] , [14] . However, our results indicate, together with other records [4] , that the latitudinal displacement of the southernmost position of the ITCZ over the last termination was not solely controlled by the scale and intensity of northern cooling/warming events. The weakest tropical convection, resulting in dry conditions, characterizes HS1 in Northern Hemisphere SE Asian records [15] , [16] . In contrast, there is evidence for sustained precipitation in the Flores Sea area during HS1 from speleothem δ 18 O (ref. 17 ) and from 232 Th flux records as a proxy for detrital riverine input [18] . However, our records from the Timor Strait do not indicate substantially increased precipitation at this time ( Fig. 2 ), suggesting that the southernmost extension of the ITCZ during HS1 was probably relatively close to its present-day position. The similarity between these two periods can be partly explained by the fact that, at the beginning of HS1, precessional summer insolation forcing was much stronger in the Southern Hemisphere than in the Northern Hemisphere, as it is the case today [19] . However, the ITCZ may have been locked into a more equatorial position by the huge exposed landmasses in the centre of the Indonesian Archipelago, when the sea level was still substantially lower. During the YD and earliest Holocene, the Australian monsoon intensified and the ITCZ shifted further south than during HS1, although Northern Hemisphere cooling was less pronounced [3] . We relate the extended southward deflection of the ITCZ austral summer position during the YD to intensification of the Pilbara heat low-pressure cells through enhanced greenhouse forcing associated with the major deglacial atmospheric CO 2 rise between ~12.8 and 11 ka (refs 3 , 5 ). In contrast, northward shifts of the ITCZ during periods of Northern Hemisphere warming and Southern Hemisphere cooling, such as the B–A/ACR and middle Holocene (~7–5 ka), led to intensified dry trade winds, with enhanced dust fluxes and prolonged droughts over NW Australia and Timor. Interestingly, unusually wet conditions were recorded during the B-A/ACR off South Java, at a more northwesterly location than our sites [14] ( Fig. 3 ), which is subject to more intense cross-equatorial moisture transport from the Northern Hemisphere. Together with our data, these results indicate that the southern limit of the austral summer convective rain belt remained close to Java and exerted no major influence over NW Australia and the southern Timor Sea during the B-A/ACR ( Fig. 4 ). 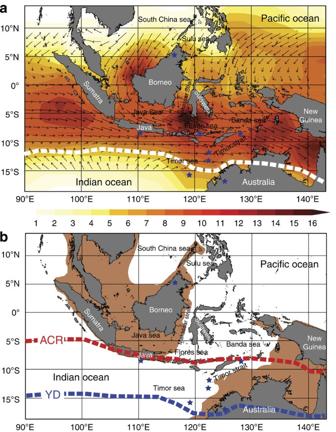Figure 4: Hypothesized deglacial displacement of the Australian monsoonal rain belt. (a) Present-day austral summer monsoon winds (arrows) and precipitation (shading; mm per day) over the Indonesian archipelago and NW Australia. Climatological summer mean precipitation (mm per day) is from climate prediction center (CPC) Merged Analysis of Precipitation 1979–2000 data52. Austral summer wind trajectories (averaged for February from 2000 to 2004)14indicate present-day areas of strong cross-equatorial flow. Southern limit of the rain belt is indicated by a white dashed line. Location of marine cores and speleothem sites are indicated by blue stars. (b) Tentative positions of the southern limit of the rain belt during the Antarctic cold reversal (ACR) and Younger Dryas (YD) are indicated by red and blue dashed lines. Brown-shaded area indicates exposed land during the Last Glacial Maximum sea-level lowstand (120 m isobath). Figure 4: Hypothesized deglacial displacement of the Australian monsoonal rain belt. ( a ) Present-day austral summer monsoon winds (arrows) and precipitation (shading; mm per day) over the Indonesian archipelago and NW Australia. Climatological summer mean precipitation (mm per day) is from climate prediction center (CPC) Merged Analysis of Precipitation 1979–2000 data [52] . Austral summer wind trajectories (averaged for February from 2000 to 2004) [14] indicate present-day areas of strong cross-equatorial flow. Southern limit of the rain belt is indicated by a white dashed line. Location of marine cores and speleothem sites are indicated by blue stars. ( b ) Tentative positions of the southern limit of the rain belt during the Antarctic cold reversal (ACR) and Younger Dryas (YD) are indicated by red and blue dashed lines. Brown-shaded area indicates exposed land during the Last Glacial Maximum sea-level lowstand (120 m isobath). Full size image The onset of intensified monsoonal precipitation exhibits a distinct NE–SW gradient through the region, occurring between ~14–15 ka in the Banda Sea [20] , at 13.4 ±0.3 ka in the Timor Strait (Core SO185-18460, Fig. 2 ), and at 11.6–13.0 ka offshore NW Australia (Cores SO185-18506, MD01-2378 and SO185-18479, Fig. 2 ). Biogenic and terrigenous proxy records in a core from the northwestern Timor Sea (off South Java), located below the present South Java Current initially indicated that dry conditions with weak monsoonal rainfall and intensified SE trades persisted until ~12 ka at that location [21] . However, recent investigations in the same area revealed a more complex pattern with an earlier onset of wet monsoon conditions during the B–A (~15–13 ka), interrupted by a brief period of intensified trade winds and dry conditions during the YD (~13–12 ka) before a second sustained increase from ~12 ka onwards [14] ( Fig. 3 ). This delayed increase is also evident in Flores speleothem records [22] ( Fig. 3 ), which are exposed to a more direct atmospheric connection to Northern Hemisphere climate along the main track of the NW monsoon. A plausible explanation for the differential onset of the Australian monsoon registered in our suite of cores and in the Banda Sea record [20] is the massive change in landmass exposure through the deglacial sea-level rise. The early monsoon onset in the eastern part of the Timor Strait and Banda Sea coincided with Meltwater Pulse 1A, which led to the flooding of Sundaland (14.6–14.3 ka) [23] . A similar mechanism has been recently proposed for the strong intensification of monsoonal rainfall over Flores at ~9.5 ka (ref. 24 ). The disappearance of a large exposed land mass probably resulted in both enhanced atmospheric cross-equatorial flow of wind surges from the South China Sea and intensified tropical convection and moisture supply over the region during austral summer [25] . These changes in land exposure were probably less significant over the Indian Ocean region, where sea-level induced changes in land–ocean configuration were restricted to the NW Australian shelf and had no influence on moisture supply along the monsoonal pathway ( Fig. 4 ). Numerical simulations support that the ITCZ over the eastern Indian Ocean sector and over the Australian continent exhibit different responses to insolation forcing [26] . However, further work is required to elucidate regional rainfall-distribution patterns during deglacial warming and sea-level rise, and to tease out relationships to forcing mechanisms and amplifying feedbacks. Our results lead to two important conclusions concerning the processes controlling the evolution of the Australian monsoon over the last glacial termination: (1) the intensification of the Australian monsoon following the ACR paralleled Southern Hemisphere warming; we speculate that intensification of the NW Australian Pilbara heat low through enhanced greenhouse forcing accentuated the southward pull of the ITCZ, thus controlling the spatial and temporal evolution of the monsoon; (2) sea-level and sea surface temperature related land–sea interactions over the Indonesian–Australian Maritime Continent altered water vapour and heat take-up by the atmosphere, as well as cross-equatorial moisture transfer, imparting a distinct spatial asymmetry to the onset and development of the monsoon through time. Chronology The chronologies of Cores SO185-18506, SO185-18579 and SO185-18460 are based on AMS 14 C dating of the surface-dwelling foraminifer Globigerinoides ruber supplemented by two oxygen-isotope tie-points over the LGM part of the record ( Supplementary Fig. 10 ; Supplementary Tables 2 and 3 ). For Core MD01-2378, we used published AMS 14 C and stable isotope data [27] , [28] , [29] , [30] ( Supplementary Tables 2 and 3 ). About 800–1,500 well-preserved tests of G. ruber were picked from the >250-μm-size fraction. AMS 14 C dating was performed at the Leibniz Laboratory, Kiel University, following the protocol described in refs 31 , 32 , except for the top sample of Core SO185-18506, which was dated at the Australian Nuclear Science and Technology Organisation, Menai, Australia (ANSTO code OZJ355). Conventional ages were converted to calendar ages following the protocol detailed in ref. 33 . We applied consistent marine reservoir age corrections of 400 years (ref. 34 ). However, the assumption of constant marine reservoir ages is problematic for the LGM, and the calibrated AMS 14 C dates older than 18 ka should be considered minimum ages [30] , [35] . An interpolated curve was fitted through the AMS 14 C data points using a Stineman function (interpolate function in KaleidaGraph) ( Supplementary Fig. 10 ). This function fits a curve that passes through the data points and matches the slopes at these points, without producing spurious results near changes of the slope. For Core MD01-2378, the function additionally has a geometric weight applied to the current point and ±10% of the data range (smooth function in Kaleidagraph), which reduces the effect of individual outliers. The resulting interpolated/smoothed curves were then sampled at intervals corresponding to XRF scanner data points (1 cm for Cores MD01-2378, SO185-18460 and SO185-18579; 0.2 cm for core SO185-18506). XRF-scanner proxy data for riverine runoff and aeolian dust Elemental composition was analysed using the second-generation AVAATECH XRF core scanners [36] at MARUM, University of Bremen and at IfG, Kiel University. XRF scanner data were collected every 1 cm (Cores MD01-2378, SO185-18460 and SO185-18579) or every 0.2 cm (Core SO185-18506) over a 1-cm 2 area with a downcore slit size of 10 mm using generator settings of 10 and 50 kV, a current of 0.25 and 1.0 mA and a sampling time of 30 s directly at the split core surface of the archive half. The split core surface for the cores was covered with a 4-μm-thin SPEXCerti Prep Ultralene1 foil to avoid contamination of the XRF measurement unit and desiccation of the sediment. The data reported here were acquired using a XR-100CR detector from Amptek and an Oxford Instruments 50W XTF5011 X-Ray tube with rhodium (Rh) target material. Raw data spectra were processed by the analysis of X-ray spectra with the Iterative Least square software (WIN AXIL) package from Canberra Eurisys. Results are reported in the natural logarithms of elemental ratios, which provide the most easily interpretable signals of relative changes in chemical composition downcore and minimize the risk of measurement artefacts from variable signal intensities and matrix effects [37] . We used the elements Al and K as proxies for the terrigenous-derived sediment-component, mainly originating from riverine transport into the Timor Sea from the NW Australian continent (Cores SO185-18506, SO185-18579 and MD01-2378) and for the sediment component mainly originating from riverine transport into the northern margin of the Timor Strait from Timor, the southern Moluku and other Indonesian islands (Core SO185-18460). We normalized these records against Ca, derived from the biogenic carbonate of a marine plankton. This approach is commonly used in carbonate-rich environments, where no indication of carbonate dissolution can be detected, for example, see refs 14 , 38 . Carbonate is the dominant component in the NW Australian cores (that is, varying between 62 and 72 weight % in Core SO185-18506, Supplementary Fig. 4 ). There is no clear relationship between increases or decreases in carbonate percentages (reflected in the XRF-scanner ln(K/Ca) records, and changes in sedimentation rates ( Supplementary Fig. 4 ), which would be expected if fluctuations in carbonate production/dissolution were the main factors controlling the clay-carbonate ratio in our cores. To further evaluate a possible bias of the Ca-normalized variability of terrigenous elements, we additionally normalized against Ba ( Supplementary Fig. 5 ), which is related to particulate organic matter and/or the precipitation of barite by marine bacteria [39] , [40] and, thus, has no direct relation to carbonate flux. In previous records from the NW Australian margin, CaO 3 and organic productivity indicators such as C org and chlorins did not show any positive correlation [41] (Core MD01-2378). Thus, we conclude that the consistent behaviour of terrigenous elements normalized against Ca or Ba ( Supplementary Fig. 5 ) indicate that fluctuations in the Ca-normalized terrigenous elemental curves are caused by fluctuations in terrigenous input rather than changing marine carbonate production/dissolution. Differences in the abundance of Zr, Ti, Fe, Al and K reflect the composition, grain size and transport pathway of terrigenous particles, since potassium and aluminium occur preferentially in river-transported fine-grained clay, whereas larger and/or heavier wind-blown grains from the Australian desert have relatively high Zr, Ti and Fe values. Titanium and zirconium are the main components of heavy minerals such as rutile and zircon, which are subject to sorting and preferential settling close to river mouths and on the continental shelf [42] , thus mainly reflecting aeolian dust transported material at distal locations. Iron oxides as discontinuous red coatings on quartz grains form an important pigmenting component of sand samples from the Australian deserts and occur in aeolian deposits in addition to iron-rich minerals (goethite and haematite) from soils of the Australian arid zones [43] , [44] , [45] . XRF-scanner-derived sedimentary Fe content has been previously used as a proxy of dust input and related wind strength in marine sediments off southern Australia [46] . Statistical change-point estimation To quantify change points, we fitted a continuous, piecewise-linear regression model, denoted as ‘ramp’ [47] to the data. The fitting procedure combines an ordinary least-squares criterion with a brute-force search for all posssible change-point times from the set of data time points. The selected fit intervals are given in Supplementary Table 1 ; Supplementary Figs 7 and 8 . Graphical regression residual analysis attested in all cases that the ramp is a suitable model for the change. In a few cases, where change points were on the fit-interval boundary, the results should be interpreted with caution. To determine the statistical uncertainty for estimated change points, we performed computing-intensive block bootstrap resampling [8] . The bootstrap (resampling from the residuals) provides robustness against violations of distributional assumptions. The resampling was carried out blockwise, with a block length determined by data size and the strength of autocorrelation (ref. 8 : equation 3.28); this procedure provides robustness against the presence of autocorrelation in the time series. The number of resamples (on which the ramp fitting is repeated each time) is 2,000. The given 1-sigma error ( Supplementary Table 1 ; Supplementary Figs 7 and 8 ) is the s.d. over the 2,000 copies of simulated start or end timing values. The software RAMPFIT [47] was adapted to perform block bootstrap resampling (RAMPFITc). RAMPFITc is available freely at http://www.climate-risk-analysis.com . How to cite this article : Kuhnt, W. et al . Southern Hemisphere control on Australian monsoon variability during the late deglaciation and Holocene. Nat. Commun. 6:5916 doi: 10.1038/ncomms6916 (2015).